Silicon-based broadband antenna for high responsivity and polarization-insensitive photodetection at telecommunication wavelengths Although the concept of using local surface plasmon resonance based nanoantenna for photodetection well below the semiconductor band edge has been demonstrated previously, the nature of local surface plasmon resonance based devices cannot meet many requirements of photodetection applications. Here we propose the concept of deep-trench/thin-metal (DTTM) active antenna that take advantage of surface plasmon resonance phenomena, three-dimensional cavity effects, and large-area metal/semiconductor junctions to effectively generate and collect hot electrons arising from plasmon decay and, thereby, increase photocurrent. The DTTM-based devices exhibited superior photoelectron conversion ability and high degrees of detection linearity under infrared light of both low and high intensity. Therefore, these DTTM-based devices have the attractive properties of high responsivity, extremely low power consumption, and polarization-insensitive detection over a broad bandwidth, suggesting great potential for use in photodetection and on-chip Si photonics in many applications of telecommunication fields. Plasmonic nanostructures can be used to increase the harvesting of incident light and enhance the performance of various optoelectronic devices [1] , [2] , [3] , [4] , [5] , [6] . Conventionally, these metallic nanostructures are placed on or close to the active region of the device, thereby generating a strong electric field within the near field and increasing the photon density of states to modify or enhance the device performance [7] . The interaction of light with nanostructured metals can cause the near-field optical field to increase by several orders of magnitude relative to the incident light. Many types of plasmonic metal nanostructures have been developed, including nano-apertures [8] , nanoparticles, and nanoantennas [7] , [9] , [10] . The use of metallic nanostructures as an optical antenna on a semiconductor material, such as silicon (Si), germanium (Ge) [8] , [10] , and graphene [11] , [12] , can enhance the photoresponse of a device, mainly from the strong near-field optical intensity around the metallic nanostructures further increasing the absorption of light in the semiconductors. Furthermore, the concept of using diodes to directly rectify the current induced by antenna structures for photodetection also has been reported [13] , [14] . These devices were typically using the micron-size antennas composed by a metal-insulator-metal (MIM) structure to guide surface plasmons into the high speed diodes for light detection in the IR regime. In great contrast with previous studies, Knight et al. [7] recently proposed a distinguished concept of using an active antenna for photodetection well below the band edge of the semiconductor material. The novel concept was to combine the functions of a nanoantenna and a photodiode within the same structure, which they called an ‘active’ optical antenna. They demonstrated active antennas [7] on Si substrates that caused the hot carriers arising from surface plasmon decay to generate photocurrent directly for the detection of infrared ray (IR) light in optical telecommunication regimes. This method overcomes the native limitations of Si, which possesses a band gap energy ( ca. 1.12 eV) that limits the ability to convert light below the band edge of Si. Moreover, a photocurrent can be generated when the photon energy is only slightly higher than the Schottky barrier height [15] . Therefore, Si-based photodetectors can not only detect photons well below the band edge of Si but also provide great potential for the on-chip silicon photonics [16] , [17] , [18] , [19] . Typically, exploiting the properties of localized surface plasmons in the visible or near-infrared ray (NIR) regime requires local surface plasmon resonance (LSPR)-based antennas to have dimensions in the range from approximately 50 to 250 nm [20] . Therefore, the nanoantennas are generally fabricated using focus ion beam (FIB) or electron beam lithography (EBL) manufacturing processes, both of which are complicated and expensive. Therefore, an essential challenge remains to develop a new active antenna structure that can dramatically enhance the photoresponsivity of the semiconductor to well below the band edge. Furthermore, with consideration of a practical photodetection technology, the antennas must meet the following requirements: high responsivity and detectivity, simple fabrication, identical photoresponse toward different polarization states of light, and the capability of photodetection over a broad bandwidth. The nature of LSPR and the properties of metal gratings mean, however, that devices based on these structures must intrinsically possess only narrow-bandwidth photoresponses and limited detection of certain polarizations of light [7] , [21] . In this study, we propose a new concept for the development of three-dimensional (3D) antennas: deep-trench/thin-metal (DTTM) active antenna structures that enhance the photoresponsivity of the semiconductor well below the band edge. The DTTM structure proposed herein exploits both surface plasmon resonance (SPR) and 3D cavity effects to effectively collect hot electrons arising from plasmon decay and, thereby, directly generate a photocurrent under zero bias voltage. This DTTM-based strategy not only extends the band edge of Si into the IR regime but also broadens the bandwidth of the photoresponse with polarization-insensitive detection. Design of the DTTM active antenna-based devices In recent years, there has been considerable interest in the use of plasmonic structures to enhance the performance of optoelectronic devices. These plasmonic structures can confine the electric field within near fields and generate ‘hot’ and energetic electron through plasmon decay. This concept can also be achieved from metallic active antenna structures prepared on Si surfaces, where metal–Si Schottky barriers are formed. 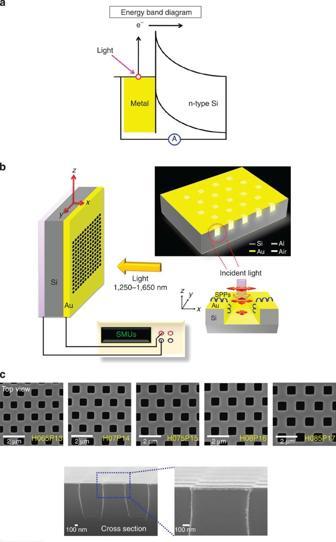Figure 1: DTTM–Schottky photodetector. A plasmonic device possessing the DTTM active antenna structure for photodetection well below the semiconductor band edge. (a) Energy band diagram for plasmonically driven ‘hot’ electrons over a metal–semiconductor Schottky barrier. (b) Schematic representation of the electrical measurement set-up and proposed DTTM active antenna structure on a Si-based device. (c) Top-view and cross-sectional scanning electron microscopy images of DTTM structures on Si substrates. Figure 1a provides a schematic representation of the energy band diagram of a metal–Si interface. When the surface of the metal is illuminated with light, the active antennas can generate and inject hot electrons into the Si over the Schottky barrier, thereby contributing to the photocurrent. By using the strategy of an active antenna, the generation of the photocurrent is no longer limited to photon energies greater than the band gap energy of the semiconductor materials, but instead to photon energies just above the Schottky barrier height. Therefore, a device featuring an active antenna structure is capable of detecting light with photon energies well below the band gap energy of the semiconductor. Figure 1: DTTM–Schottky photodetector. A plasmonic device possessing the DTTM active antenna structure for photodetection well below the semiconductor band edge. ( a ) Energy band diagram for plasmonically driven ‘hot’ electrons over a metal–semiconductor Schottky barrier. ( b ) Schematic representation of the electrical measurement set-up and proposed DTTM active antenna structure on a Si-based device. ( c ) Top-view and cross-sectional scanning electron microscopy images of DTTM structures on Si substrates. Full size image In this paper, we propose the concept of electric field enhancement through use of active antenna structures exploiting both SPR and 3D cavity effects. We demonstrate the photodetection ability of 3D deep-trench-based active antenna structures, which effectively generate ‘hot’ electron through plasmon decay to obtain the photocurrent directly with a broad bandwidth. Figure 1b displays a schematic representation of the measurement set-up and the proposed DTTM structure. We illuminated the DTTM-based devices with tungsten lamp and a tunable laser in the IR regime. We extracted the current–voltage data using a digital source metre and measured the responsivity with respect to the wavelength of the incident light. The inset to Fig. 1b displays a DTTM structure, based on a thin Au film, prepared on the surface of a Si substrate. The DTTM structures exploited both SPR and cavity effects, allowing the wavelength of the resonances to be adjusted by varying the diameter, depth and period of the deep-trench structures. Furthermore, the large area of Schottky junction in deep trenches is a very important feature for increasing the conversion efficiency of active antenna-based photodetection. In previous study, the vertical Schottky interfaces in nanoantenna-based devices were demonstrated having a great contribution to the photo-response [22] . Accordingly, the Au/Si interfaces in the deep trenches sufficiently construct the 3D Schottky interfaces with large area on both the surface and vertical sides of the DTTM structures. In addition, the area of vertical Schottky interfaces in the DTTM structures is larger than those on the surface. Therefore, the proposed DTTM structures would be expected to provide both the enhancement of optical absorbance and the improvement of extraction of hot electrons. Figure 1c displays scanning electron microscopy images of DTTM structures of various diameters and periods uniformly and deeply etched into the Si surface in a hexagonal arrangement. Herein, we label the plasmonic devices in terms of their distinct dimensions (diameter and period) in Table 1 ; for example, the device featuring a DTTM structure having a diameter of 0.65 μm and a period of 1.3 μm is named ‘H065P13’. The ratio of the diameter to the period in the DTTM structures was set at 1:2; the other DTTM structures in the devices are named H07P14, H075P15, H08P16 and H085P17. Furthermore, the cross-sectional images reveal that the Au layers provided good coverage, according to the surface profiles of the deep trenches on the Si surfaces. Therefore, we expected the DTTM-based active antenna structures would provide not only strong electric fields within the near field but also metal–semiconductor (Au/Si) junctions with very large surface areas to propose the concept of electric field enhancement through use of active antenna structures exploiting both SPR and 3D cavity effects. Table 1 The labels of the DTTM-based devices in terms of distinct dimensions. Full size table Optical behaviours of the DTTM active antenna structure To increase the photoresponse dramatically below the band gap of the semiconductor, we investigated various types of plasmonic structures using the 3D finite-difference time-domain (3D–FDTD) method. When choosing a design for the active antennas, we considered the ease of fabrication and the strengths of absorption and electric fields around the metal–semiconductor junction. As displayed in Fig. 2a , we compared four types of active antenna structures on Si: metal nanorod (nanoantenna) arrays, metal dot arrays, metal hole arrays and DTTM arrays. The dimensions of a nanoantenna displaying LSPR properties are generally in the range from ~10 to 100 nm. As displayed in Fig. 2a , in the study of Knight et al. [7] the width and length of the nanoantenna arrays were 50 nm and 116 nm, respectively. Such nanoscale-active antennas are prepared using complicated FIB or EBL techniques. Therefore, to decrease the difficulty of the fabrication processes, we wished to increase the dimensions of the nanoantennas to >0.5 μm, allowing their preparation rapidly and readily through conventional optical lithography. In Fig. 2a , the width and period of the square dot arrays are 0.65 μm and 1.3 μm, respectively. By increasing the dimensions of the antenna to the half-micrometre scale, we expected these larger Au dot arrays to lose their LSPR behaviour, resulting in weak electromagnetic fields around the metal dot arrays. In previous studies, sub-micrometre metal hole arrays have exhibited extraordinary optical transmission phenomena with high electromagnetic fields [6] . As displayed in Fig. 2a , the width and period of the hole arrays were also 0.65 μm and 1.3 μm, respectively. The degree of near-field enhancement in these holes was, however, still much lower than that around the nanoantennas having LSPR properties. Therefore, in this study we proposed a new structure to take advantage simultaneously of the SPR phenomenon of hole arrays and the large near-field enhancements in cavities. As displayed in Fig. 2a , the width, period and depth of the DTTM arrays were 0.65 μm, 1.3 μm and 1.2 μm, respectively. This deep-trench structure featuring periodic metal trenches can generate surface plasmon polariton (SPP) waves. Moreover, the deep-trench structure can provide 3D cavities to confine the propagation of SPP waves. Therefore, we expected to observe an electromagnetic field with high intensity around the DTTM antenna structures. 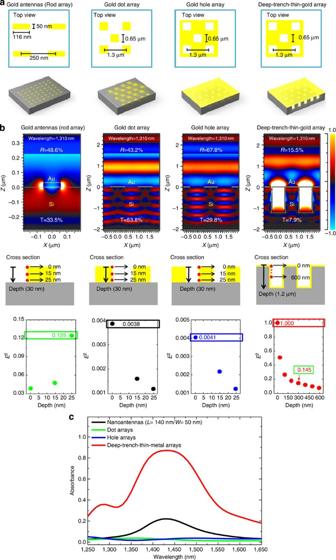Figure 2: Optical behaviours of various types of active antenna structures. (a) The presence of the antenna structures are nanoantennas, dot arrays, hole arrays and DTTM arrays. The thickness of the Au film in each structure was 30 nm and the detail dimensions were described. (b) A plane wave having a wavelength of 1,310 nm was propagated above the air-structured metal interface to the Si substrate. All the squares of the electric field amplitudes (|E2|) at distinct depths have been normalized to the highest value of |E2|, which was generated at the surface of the DTTM arrays. Compared with other types of antenna structures, the DTTM arrays provided the strongest optical electric field intensity within its near field. Moreover, the DTTM arrays exhibited high electric field strength in the large volume of the cavity and also around the large area of the air–Au interface. (c) Corresponding simulated absorption spectra of the four types of antenna structures. Among them, the DTTM arrays exhibited the largest absorption in the broadband regime. Figure 2: Optical behaviours of various types of active antenna structures. ( a ) The presence of the antenna structures are nanoantennas, dot arrays, hole arrays and DTTM arrays. The thickness of the Au film in each structure was 30 nm and the detail dimensions were described. ( b ) A plane wave having a wavelength of 1,310 nm was propagated above the air-structured metal interface to the Si substrate. All the squares of the electric field amplitudes (| E 2 |) at distinct depths have been normalized to the highest value of | E 2 |, which was generated at the surface of the DTTM arrays. Compared with other types of antenna structures, the DTTM arrays provided the strongest optical electric field intensity within its near field. Moreover, the DTTM arrays exhibited high electric field strength in the large volume of the cavity and also around the large area of the air–Au interface. ( c ) Corresponding simulated absorption spectra of the four types of antenna structures. Among them, the DTTM arrays exhibited the largest absorption in the broadband regime. Full size image As displayed in Fig. 2b , we set plane waves (wavelength: 1,310 nm) propagating above the four types of active antenna structures on Si substrates. To further study the optical behaviour of the incident light through the different antenna structures, we set up three detectors on the structure’s (nanoantennas and dot/hole arrays) sidewall (0 nm, 15 nm, 25 nm, respectively, below the top surface of Au); additionally, we set up eight detectors on the sidewall of trench structure (0 nm, 30 nm, 100 nm, 200 nm, 300 nm, 400 nm, 500 nm and 600 nm, respectively, below the top surface of DTTM arrays). In the simulations, we set the thickness of the Au film in each antenna structure at 30 nm and obtained the optical constants of Si and Au from the literature [23] . Figure 2b displays the electric field distributions generated from incident light passing through the four types of antenna structures. We found that the DTTM arrays provided the strongest electric fields within the near field around the air–Au interface. In Fig. 2b , we normalized all of the values of the square of the electric field amplitude (| E 2 |) at distinct positions to the strongest value of | E 2 | generated around the surface of the DTTM arrays. At first, we considered the previously reported nanoantenna arrays; this structure with LSPR properties did indeed enhance the absorption of the metal and provided large electric fields in sub-wavelength regimes. The value of | E 2 | of that nanoantenna remained; however, approximately one order of magnitude lower than that of the DTTM arrays proposed in this study. Furthermore, we found that dot and hole array structures having the same dimensions (period, width and thickness of Au layers) as the DTTM structure provided very low electric field intensities relative to those of the DTTM antenna structure. The deep-trench antenna structure displayed superior light trapping properties, with values of | E 2 | near the air–Au interface approximately two orders of magnitude higher than those of the dot and hole arrays. Furthermore, the DTTM-based active antenna structure can exploit both SPR and cavity effects. The generation of an SPP wave arises from the coupling of light to the surface plasmon excitation of a periodic metal structure. The generated SPP waves propagate into the cavity of the DTTM structure and then decay gradually to increase the momentum of hot electrons. Therefore, the resulting near-field electric field in the cavity of a DTTM structure can be one order to two orders of magnitude higher than those in the other three types of antenna structures. Figure 2b also reveals that the electric field intensity in the cavity 0.3 μm under the surface of the DTTM structure was still higher than the highest electric field intensity of the nanoantenna structure. Most importantly, the effective area of the metal–semiconductor (Au–Si) interface within the high-electric-field regime in the DTTM-based active antenna was much larger than those of other antenna structures. Figure 2c displays the absorbance spectra of the four types of antenna structures, as simulated using the 3D-FDTD method. The absorbance spectra reveal that the nanoantenna and the DTTM-based active antennas both featured absorptions at a wavelength of 1,420 nm. The peak value of this absorbance for the DTTM arrays (88%) was, however, four times and one order of magnitude larger than those of the nanoantennas and dot/hole arrays, respectively. Moreover, compared with the other antenna structures, the DTTM array-based active antenna exhibited the largest absorption in the broadband regime. With the goal of detecting light having photon energy below the semiconductor band edge, it was necessary to increase the number of ‘hot’ electron/hole pairs generated upon light absorption by the active antennas formed from the metal structures. Therefore, we expected the DTTM arrays to exhibit the highest plasmonic-induced photoresponses over broad bandwidth regimes. The DTTM-based active antenna structure appeared to possess the following superior properties: high electric field intensity over a large volume within the near field of the antenna structure; high absorption of the active antenna; working over broad wavelength range and a large-area metal–Si interface. Therefore, we suggested that the DTTM structure would be appropriate for photodetection in IR regimes, well below the band edge of Si. Furthermore, a practical photodetection technology must meet the following criteria: high responsivity and detectivity; identical photoresponses toward different polarization states of light [24] ; simple fabrication and photodetection capability over a broad bandwidth [1] , [3] . In previous studies, LSPR-based active nanoantennas and metal grating-based antenna structures have generated hot electrons for photodetection in the IR regime [7] , [21] . Nevertheless, the intrinsic properties of LSPR or a metal grating imply that a device based on nanoantennas or metal gratings must display a photoresponse with only a narrow bandwidth and must have limited ability to detect certain polarization states of light. As displayed in Fig. 3 , we applied the 3D-FDTD method to simulate the optical behaviour of a nanoantenna and a DTTM-based active antenna illuminated under distinct wavelengths and different polarization states of light. We first considered a previously reported nanoantenna structure having a length of 140 nm and a width of 50 nm. As displayed in Fig. 3a , the nanoantenna structure was optimized for large LSPR phenomena for x -polarized light at a wavelength of 1,420 nm. The incident light was x -polarized with transverse polarization of the electric field to the orientation of the long axis of the nanoantenna. For x polarization of incident light, the nanoantenna featured large electric field intensity at a wavelength of 1,420 nm. When we shifted the wavelength of incident light away from the plasmonic resonance wavelength to 1,310 or 1,550 nm, however, the electric field intensity around the structure decreased significantly. The electric field distributions of the nanoantenna when illuminated at distinct wavelengths were obviously different, clearly revealing that the wavelength of incident light would be critical for the generation of LSPR-induced hot electrons in active nanoantenna-based photodetectors. Only a narrow bandwidth of incident light could be used to generate the plasmonic response and hot electrons in such a device. 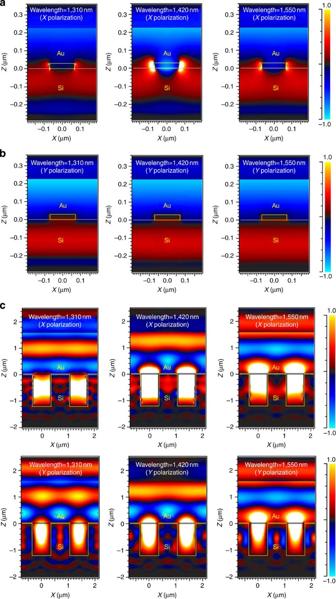Figure 3: Polarization-insensitive photodetection. Optical behaviour of nanoantenna (Lrod=140 nm;Wrod=50 nm) and DTTM (H07P14) arrays simulated using the 3D-FDTD method to investigate the effects of incident light with different polarization states and distinct wavelengths on the antennas. (a) Forx-polarized light, the nanoantenna provided large electric field intensities at 1,420 nm, but the near-field intensities decreased dramatically as the wavelength moved away from the LSPR wavelength. (b) Fory-polarized light, the nanoantenna did not reveal any plasmonic responses at wavelengths of 1,310, 1,420 or 1,550 nm. (c) The DTTM active antenna displayed high electric field intensities around the antenna structures at distinct wavelengths, regardless of the polarization of the incident light. Figure 3: Polarization-insensitive photodetection. Optical behaviour of nanoantenna ( L rod =140 nm; W rod =50 nm) and DTTM (H07P14) arrays simulated using the 3D-FDTD method to investigate the effects of incident light with different polarization states and distinct wavelengths on the antennas. ( a ) For x -polarized light, the nanoantenna provided large electric field intensities at 1,420 nm, but the near-field intensities decreased dramatically as the wavelength moved away from the LSPR wavelength. ( b ) For y -polarized light, the nanoantenna did not reveal any plasmonic responses at wavelengths of 1,310, 1,420 or 1,550 nm. ( c ) The DTTM active antenna displayed high electric field intensities around the antenna structures at distinct wavelengths, regardless of the polarization of the incident light. Full size image The nanoantenna structure is also very sensitive to the polarization state of the incident light. As displayed in Fig. 3b , the nanoantenna structure ( L rod =140 nm; W rod =50 nm) did not display any localized plasmonic resonance phenomena when applying y -polarized incident light. We found that the intensity of the electric field around the structures was not be enhanced when the incident light was y -polarized for wavelengths of 1,310, 1,420 or 1,550 nm. Obviously, the nanoantenna-based device exhibited significant selectivity for the polarization state of light, thereby seriously limiting the practical application of nanoantennas for photodetection. The LSPR-based active nanoantennas can detect light only with a certain polarization and within a narrow spectral window. Therefore, this nanoantenna structure would not be suitable for the practical photodetection of randomly polarized, broadband incident light. In contrast, the DTTM structure proposed in this study was not selective for the polarization state of light and exhibited broadband photodetection capability. As displayed in Fig. 3c , the DTTM (H07P14) structure with hexagonal symmetry meant that, no matter whether the light was x - or y -polarized, the deep-trench arrays provided large electric field intensities within the near field at a wavelength of 1,420 nm. Furthermore, the DTTM structure exploited both SPR and cavity effects, not only at a wavelength of 1,420 nm but also at 1,310 and 1,550 nm, providing large electric field intensities within the near field around the antenna structures. Therefore, we expected active antennas based on deep-trench arrays to have great potential for applications in broadband, polarization-insensitive photodetection well below the semiconductor band edge. In this study, with regard to the simplicity of the fabrication processes and the stability of the metal, we applied a single-layer Au film to prepare the active antenna. Moreover, because the plasmonic-induced hot electrons were generated directly in the Au layer, we could focus on the optical behaviours of DTTM antenna structures that would directly affect the photoresponse of devices. In addition, the stability of the metal should also be taken into consideration. Even though a Ti–Si or Ag–Si interface might provide a higher quantum transmission probability than that of an Au–Si interface, Ti and Ag are much more prone to oxidation in air than is Au. In this study, we prepared a DTTM-based active antenna structure that featured only a single-layer Au antenna. Furthermore, we employed the deep-trench structure, possessing excellent light trapping and hot electron generation capabilities, to overcome the much lower quantum transmission probability at the Au–Si interface, relative to that at the Ti–Si interface (see Supplementary Fig. 1 and Supplementary Note 1 ). Electrical characteristics of the DTTM active antenna-based devices Next, we measured the current–voltage performance of the DTTM-based devices for confirming the rectification of a Schttoky junction (details in Supplementary Fig. 2 ) and the photoresponsive properties of devices featuring DTTM active antennas of various sizes on the Si substrates. All of the photoresponsivity curves ( Fig. 4a ) featured higher responsivities in the shorter wavelength regime, gradually decreasing upon increasing the wavelength of the incident light. We also found that these responsivity spectra were very similar to the quantum transmission probability curves of the Au–Si interface obtained from the modified Fowler equation (see Supplementary Fig. 1 and Supplementary Note 1 ). Moreover, these response spectra exhibited a wavelength-shift in the peak responsivity upon increasing the period of the DTTM structure. Thus, the wavelengths of peak responsivity of these devices were not identical to the wavelengths of maximum absorbance simulated using the 3D-FDTD method (see Supplementary Fig. 3 and Supplementary Note 2 ). The curve reveals the gradual decrease in responsivity upon increasing the wavelength of incident light, thereby shifting the measured peak responsivity to shorter wavelength. Moreover, the experimental data reveal that even the peaks of the SPRs excited in these structures did not match in the regime between 1,250 and 1,650 nm; these devices still can exhibit high responsivity over the whole spectral regime. However, as the SPR peak of the DTTM structures is far away from the measured spectral regime (from 1,250 to 1,650 nm), the devices would reveal very low responsivities (see Supplementary Fig. 4 ). Therefore, we suggested that the SPR and 3D cavity effects both are very important for the DTTM structures. 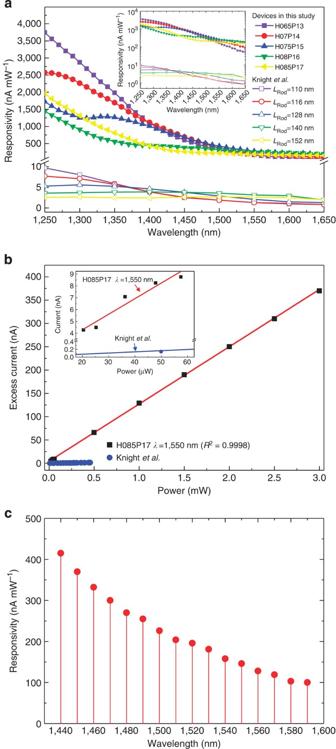Figure 4: Electrical characteristics of the DTTM active antenna-based devices. (a–c) Photoelectric characteristics of the DTTM-based devices measured under a bias voltage of 0 V. (a) Responsivity spectra of the proposed DTTM devices and of the nanoantenna-based devices reported by Knightet al.7(b) Correlation between excess current and incident light power for the DTTM-based device at a wavelength of 1,550 nm. Within the incident power range from 20.5 μW to 3 mW, the excess current of the DTTM device exhibited a linear response (R2=0.9998). (c) Distribution of the responsivity of a DTTM device at wavelengths from 1,440 to 1,590 nm when illuminated at high power density with light from a tunable laser. Figure 4: Electrical characteristics of the DTTM active antenna-based devices. ( a – c ) Photoelectric characteristics of the DTTM-based devices measured under a bias voltage of 0 V. ( a ) Responsivity spectra of the proposed DTTM devices and of the nanoantenna-based devices reported by Knight et al. [7] ( b ) Correlation between excess current and incident light power for the DTTM-based device at a wavelength of 1,550 nm. Within the incident power range from 20.5 μW to 3 mW, the excess current of the DTTM device exhibited a linear response ( R 2 =0.9998). ( c ) Distribution of the responsivity of a DTTM device at wavelengths from 1,440 to 1,590 nm when illuminated at high power density with light from a tunable laser. Full size image Figure 4b compares the measured data for nanoantenna-based devices published by Knight et al. [7] with those obtained in this study. Although the barrier height of the Au–Si interface is much higher than that of the Ti–Si interface, the responsivity of our proposed DTTM-based devices under a bias voltage of 0 V remained two or three orders of magnitude higher than those of the nanoantenna-based devices in the IR wavelength regime. Figure 4b displays the correlations between the excess current and incident power of light at the wavelength of 1,550 nm. The linear behaviour of the excess current is dominated by the conversion of incident photons into hot electrons over the range of illumination powers. The incident powers of the tunable laser light ranging from 20.5 μW to 3 mW ( ca. 6–40 μW μm −2 ), the excess current of the DTTM device also provided a high degree of linearity ( R 2 =0.9998) at a wavelength of 1,550 nm. Furthermore, the inset to Fig. 4b compares of low-intensity detection capability of the DTTM device with those of previously reported nanoantenna-based devices under the same illumination intensity. The excess current of the DTTM-based device was approximately two orders of magnitude higher than those of the nanoantenna-based devices, even though the DTTM device was operated at zero-bias voltage. We performed additional measurements to check the performance of the DTTM-based device using tunable laser under high-intensity incident light of ~40 μW μm −2 (that is, 4,000 W cm −2 ). Figure 4c reveals the broadband and high responsivities of this system toward laser light tuned in the range from 1,440 to 1,590 nm. Notably, the responsivities toward low- and high-intensity incident light were both related to the energy-dependent internal photoemission probability derived from the Fowler theory [7] . The devices comprising DTTM-based active antennas on Si also exhibited image detection capability at low levels of visible and IR light. 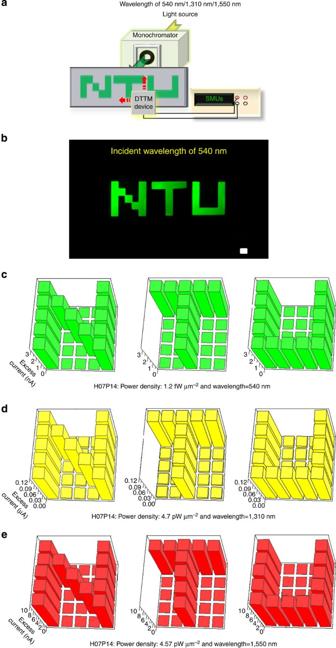Figure 5: Demonstration of detection capability. Testing image detection capability under low-intensity light at wavelengths of 540, 1,310 and 1,550 nm. (a) Schematic representation of the point-by-point scanner set-up used to test the image capture capability of DTTM active antenna-based devices. (b) Images captured by a professional digital camera under light at wavelengths of 540 nm. (c–e) Bar chart-type images provided by the H07P14-containing DTTM device under an applied bias voltage of 0 V, detected at wavelengths of (c) 540, (d) 1,310 and (e) 1,550 nm. The images were constructed based on the existence or absence of a photocurrent during the point-by-point scanning of the DTTM device. Clear images of the capitalized letters ‘NTU’ were obtained, even though the incident power density was low; for example, 4.7 pW μm−2at a wavelength of 1,310 nm and 4.57 pW μm−2at a wavelength of 1,550 nm. The scale bar (b) and the pixel size (c–e) are 5 mm. Figure 5a provides a schematic representation of the experimental set-up. By scanning the Si-based DTTM device through the slit, the photocurrent and the scan location were recorded simultaneously to obtain a distribution of photocurrents that allowed us to reconstruct an image of the letters ‘NTU.’ We used the light at an intensity of 1.2 fW μm −2 at a wavelength of 540 nm, an intensity of 4.7 pW μm −2 at a wavelength of 1,310 nm, and an intensity of 4.57 pW μm −2 at a wavelength of 1,550 nm, respectively, to investigate the DTTM device’s image detection capability. Figure 5b displays the clearly recognized image captured by the professional digital camera (Nikon D90) when the incident wavelength was 540 nm. Because of the intrinsic absorption ability of Si, the image captured is failed as the wavelengths of light are >1,200 nm. By scanning the Si-based DTTM device through the slit, the photocurrent and the scan location were recorded simultaneously to obtain a distribution of photocurrents for reconstructing an image of the letters ‘NTU’ at an intensity of 1.2 fW μm −2 at a wavelength of 540 nm ( Fig. 5c ), an intensity of 4.7 pW μm −2 at a wavelength of 1,310 nm ( Fig. 5d ) and an intensity of 4.57 pW μm −2 at a wavelength of 1,550 nm ( Fig. 5e ), respectively. Obviously, the Si-based DTTM devices displayed excellent ability for photodetection beyond the optical absorption regime of the Si material. Furthermore, the DTTM active antenna-based devices have the potential to integrate with a Si-based waveguide. Preparing the DTTM structures onto a waveguide is a good way to further enhance the responsivity of DTTM devices and easily apply the DTTM devices onto Si photonics. Thus, devices featuring DTTM-based active antennas have great potential for their high responsivity, broadband and zero-bias operation, simple fabrication and polarization-insensitive photodetection on Si at telecommunication wavelengths. Figure 5: Demonstration of detection capability. Testing image detection capability under low-intensity light at wavelengths of 540, 1,310 and 1,550 nm. ( a ) Schematic representation of the point-by-point scanner set-up used to test the image capture capability of DTTM active antenna-based devices. ( b ) Images captured by a professional digital camera under light at wavelengths of 540 nm. ( c – e ) Bar chart-type images provided by the H07P14-containing DTTM device under an applied bias voltage of 0 V, detected at wavelengths of ( c ) 540, ( d ) 1,310 and ( e ) 1,550 nm. The images were constructed based on the existence or absence of a photocurrent during the point-by-point scanning of the DTTM device. Clear images of the capitalized letters ‘NTU’ were obtained, even though the incident power density was low; for example, 4.7 pW μm −2 at a wavelength of 1,310 nm and 4.57 pW μm −2 at a wavelength of 1,550 nm. The scale bar ( b ) and the pixel size ( c – e ) are 5 mm. Full size image Knight et al. [7] proposed the novel concept of LSPR-based active nanoantennas for photodetection well below the semiconductor band edge. A practical photodetection technology must, however, meet several requirements: high responsivity, broadband detection capability, low power consumption, simple fabrication and polarization-insensitive detection. Because of the nature of LSPR, devices based on LSPR-based active nanoantennas cannot meet these requirements. In this study, we propose a new DTTM-based active antenna structure that takes advantage of SPR phenomena, 3D cavity effects and large-area metal/semiconductor junctions that effectively generate and collect hot electrons arising from plasmon decay to directly increase photocurrent. The DTTM-based strategy not only extends the band edge of Si to the IR regime but also dramatically increases the photoresponse over a broad bandwidth of light with polarization-insensitive detection. Even in the absence of any external bias voltage, the responsivity of the DTTM-based devices remained hundreds of times higher than those of LSPR-based active nanoantennas. The DTTM-based devices also displayed excellent photoelectron conversion capability, high degrees of detection linearity under light of both low ( ca. 1 pW μm −2 ) and high ( ca. 40 μW μm −2 ; that is, 4,000 W cm −2 ) intensity and image detection capability at low levels of both visible and IR light. Therefore, these DTTM-based devices possess several attractive properties—high responsivity, extremely low power consumption and polarization-insensitive detection over a broad bandwidth of light—that suggest they have great potential for use in photodetection and on-chip Si photonics in the IR and telecommunication regimes that employ mature Si technology. Sample fabrication The devices were fabricated on doped n-type Si wafers, whose doping level was ~10 15 cm −3 , grown with 100 nm of thermal oxide. The patterning process was performed using conventional I-line lithography. Before the formation of deep-trench structures in the Si substrate, the patterned sample was placed in a transformer-coupled plasma etcher to open the window on the oxide layer; furthermore, the patterned oxide could be used as an etching hard mask for deeply etching Si with the depth of ~1.2 μm. The transformer-coupled plasma is a planar, inductive source, which can achieve high density plasma operation. We could easily control the etching rate by adjusting the plasma power and gas flow rate. The conditions of dry etching for Si are described as following: chamber temperature/pressure: 65 °C/12 mT; applied power of top plate/bottom plate: 310 W/120 W; species of gas/gas flow: Cl 2 /35 sccm, HBr/125 sccm; etching rate: ~4 nm/s. After etching, the patterned Si substrate was cleaned using the standard RCA cleaning process to remove any residual photoresist and oxide. The sample was then immediately placed in a sputtering system to prevent growth of native oxide and, thereby, ensure good contact between the metal and Si. Next, a 30-nm film of Au was deposited by the sputter system to cover the deep-trench Si structure. Finally, the ohmic contact of the back electrode was deposited in a physical vapour deposition system, providing a device possessing 3D-DTTM active antennas. Device characterization A tungsten lamp (filtering wavelengths from 1,250 to 1,650 nm illuminated through a monochromator) and a high-power-intensity tunable laser (Agilent, HP 8168F; operating at wavelengths from 1,440 to 1,590 nm) were chosen as light sources for characterizing the active antenna-based devices. By tuning the monochromator, the incident light could be obtained with distinct wavelengths. The measured current–voltage data from devices with different DTTM structures were extracted using a digital source metre (Keithley 2400). The excess current, defined as the difference between the photocurrent and dark current, was obtained from the measurement data of the devices under illumination at different intensities and wavelengths of incident light. The measured photoresponsivities of the devices, with respect to the wavelength of incident light, were also obtained from the measurement data. How to cite this article: Lin, K.-T. et al. Silicon-based broadband antenna for high responsivity and polarization-insensitive photodetection at telecommunication wavelengths. Nat. Commun. 5:3288 doi: 10.1038/ncomms4288 (2014).